Oxic methanogenesis is only a minor source of lake-wide diffusive CH4emissions from lakes Determination of the contribution of oxic methanogenesis to diffusive CH 4 emissions Net production of methane in oxic waters (NOM) in the surface mixed layer (SML) is estimated as the difference between the total diffusive CH 4 emissions from the lake surface, F surf,tot , and the total flux from the sediments in the SML, F sed,tot , i.e., NOM = F surf,tot − F sed,tot . This procedure neglects processes contributing to the mass balance, e.g., vertical transport of CH 4 into the SML, but allows for a consistent comparison of the observations from Lake Hallwil and Lake Stechlin with the results derived from data of DelSontro et al. [7] . Note that the neglected processes are typically small [5] or uncertain (e.g., estimates of turbulent diffusivities in the thermocline have large uncertainty; the amount and dissolution of microbubbles were not measured in the studies considered by ref. [5] ) and are sources of CH 4 in Lake Hallwil and Lake Stechlin [5] . Our estimates are therefore upper limits of NOM. The contribution of NOM to overall diffusive CH 4 emission is defined as: NOMC = NOM/ F surf,tot . The advantage of using NOM instead of gross production of CH 4 is explained in Supplementary Note 1 . Re-evaluation of the analysis of Günthel et al. [5] : data of Donis et al. [6] from Lake Hallwil In Lake Hallwil, the contribution of oxic methanogenesis to overall diffusive CH 4 emissions has been estimated to be 90% [6] or 63–83% [5] , but we show here that NOMC ~ 17%. In the mass balance of the SML extending from 0 to 5 m water depth [5] , [6] , Günthel et al. [5] used an average sediment flux of F sed = 1.75 mmol m − 2 day −1 , averaging flux estimates of Donis et al. [6] from two sediment cores, one collected at 3 m and the other at 7 m water depth. The δ 13 C of the CH 4 in the pore water of these two cores differ substantially [6] , indicating differences in production and oxidation of CH 4 between the sediments in the SML and at 7 m water depth. The estimate of F sed in the SML should therefore be based on the core collected at 3 m water depth. Using the approach of Donis et al. [6] , the correct F sed derived from the data of this core is F sed = 2.8 mmol m − 2 day −1 (Peeters et al. [9] , see Supplementary Note 2.1 for details). Günthel et al. [5] and Donis et al. [6] apparently have erroneously used gas transfer coefficients instead of proper CH 4 fluxes to calculate emissions. This conclusion is demonstrated by the perfect agreement between the values published erroneously as CH 4 fluxes, F surf , by Günthel et al. 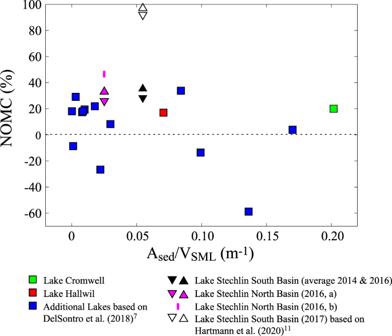Fig. 1: The contribution of net oxic methane production to the diffusive CH4emission from lakes. The contribution of net oxic methane production to the diffusive CH4emission, NOMC, was calculated in the different lakes from the surface CH4flux,Fsurf, and the methane flux from the sediments,Fsed, obtained from different data sources: Lake Hallwil (Supplementary Table1):Fsurffrom the “Hallwil relationship” that is based on the chamber measurements in Lake Hallwil6.Fsed, from the CH4pore water concentrations in the sediment core collected at 3 m water depth (Fsed= 2.8 mmol m−2day−1, Supplementary Table1). Lake Stechlin (Supplementary Table3): Lower and upper limits ofFsed(Fsed= 1.8 mmol m−2day−1andFsed= 2.0 mmol m−2day−1) from the re-evaluation of the mesocosm experiments (Supplementary Table2) providing upper and lower limit of NOMC, respectively (Supplementary Table3). South Basin (average 2014, 2016):Fsurffrom the “Stechlin relationship”; North Basin (2016, a):Fsurffrom chamber measurements; North Basin (2016, b)Fsurffrom chamber measurements combined with the “Stechlin relationship” for the 20 June; Lake Stechlin South Basin (2017) (Supplementary Table4):Fsedderived from CH4pore water measured in a single sediment core by ref.11, considering the CH4gradient in the top 2 cm and at 5 cm depth (Fsed= 0.08 mmol m−2day−1andFsed= 0.26 mmol m−2day−1) providing upper and lower limit of NOMC, respectively;Fsurffrom specific wind model of ref.11; Lake Cromwell: Data from ref.5. Additional Lakes (Supplementary Table5): based on the analysis of ref.7(see Supplementary Note4). The ratio between the area of the sedimentAsedand the volumeVSMLin the surface mixed layer SML,Ased/VSML, was estimated assuming a slope angle of 5° for the lake bed (Supplementary Note4). The sensitivity to the slope angle is illustrated in Supplementary Fig.5assuming a slope angle of 3°. [5] and the values of the gas transfer coefficients of CH 4 at 20 °C, k CH4 , calculated by us (Table 1 ). The values published by Donis et al. [6] as CH 4 fluxes are very similar to these k CH4 and therefore also do not represent CH 4 fluxes but gas transfer coefficients (for details, see Supplementary Note 2.2 ). Table 1 Average CH 4 surface fluxes from Lake Hallwil and gas transfer velocities. Full size table The gas transfer coefficient of CH 4 must be multiplied by the difference between the surface concentration (0.3 mmol m − 3 , ref. [6] ) and the atmospheric equilibrium concentration of CH 4 (CH 4,equ = 0.003 mmol m −3 at 20 °C [9] ), i.e. by ~0.3 mmol m −3 , to obtain F surf . F surf is therefore ~3.3 times smaller than the values of the gas transfer coefficients erroneously taken by Günthel et al. [5] and Donis et al. [6] as CH 4 fluxes (Table 1 and details in Supplementary Note 2.2 ). Donis et al. [6] and Günthel et al. [5] used values obtained from measurements with floating chambers to calculate emissions, but these values claimed to represent F surf appear to be in fact values for transfer coefficients, suggesting the same mistake as in the case of the wind models. Donis et al. [6] stated: “Average flux (April–August 2016) is equal to 0.8 ± 0.2 mmol m −2 d −1 from MacIntyre relationship for positive buoyancy and to 0.6 ± 0.3 mmol m −2 d −1 from chamber measurements. The latter, not significantly different from the wind-based relationship, was used for the mass balance”. Günthel et al. [5] , co-authored by D. Donis, claim that the “MacIntyre relationship for positive buoyancy” [10] provides an average value of 0.7 for F surf , but in fact 0.7 is the average value for k CH4 in unit m day −1 (0.7 m d −1 , see Table 1 ) and F surf for this model is 3.3 times smaller (0.21 mmol m −2 d −1 , see Table 1 ). The value by Donis et al. [6] for the MacIntyre relationship [10] is even slightly larger than 0.7 and therefore clearly incompatible with F surf but is rather a gas transfer coefficient as is obvious in the case of Günthel et al. [5] . The good agreement between the value for the gas transfer coefficient obtained from the MacIntyre model for positive buoyancy flux [10] and the values from the chamber measurements suggests that the values from the chamber measurements are not gas fluxes but also gas transfer coefficients (see Supplementary Note 2.2 for more details). Donis et al. [6] derived from their chamber measurements the wind-based model “Hallwil relationship” specifically for Lake Hallwil. The establishment of this Hallwil relationship required that Donis et al. [6] calculated gas transfer coefficients from their chamber measurements. In their Supplementary Fig. 4, Donis et al. [6] show that the values from their chamber measurements agree well with those from the Hallwil relationship (Supplementary Fig. 2 and Supplementary Note 2.2 ). Note, however, that the values for the Hallwil relationship are in fact gas transfer coefficients and not F surf , supporting that also the values from the chamber measurements represent gas transfer coefficients and not F surf (Supplementary Fig. 2 and Supplementary Note 2.2 for more details). This conclusion implies that the values from the chamber measurements by Donis et al. [6] must be multiplied by ~0.3 mmol m −3 to give proper CH 4 fluxes, which are then ~3.3 times smaller than the CH 4 fluxes used in the mass balances of refs. [5] , [6] . Because there are only four chamber measurements available for 2016 and one of them was exceptionally low (see ref. [6] and Supplementary Note 2.2 ), the Hallwil relationship is considered here to provide the most reliable estimate of the average k 600 in Lake Hallwil and therefore applied to calculate the average surface CH 4 flux for April to August 2016, i.e., F surf = 0.24 mmol m −2 d −1 (see Table 1 and Supplementary Note 2.2 ). The reliability of the Hallwil relationship was confirmed by Günthel et al. [5] and by Hartmann et al. [11] comparing different estimates of surface fluxes in the South Basin of Lake Stechlin. With F sed = 2.8 mmol m 2 day −1 and F surf = 0.24 mmol m 2 day −1 , NOM = 416 mol day −1 and the contribution of NOM to total emissions is NOMC = 17% (Supplementary Table 1 in Supplementary Note 2.3 includes also additional estimates of NOMC). The low value of NOMC suggests that most of CH 4 in the SML originates from the sediments, which is consistent with the δ 13 C isotopic composition of CH 4 in Lake Hallwil [9] . The uppermost CH 4 in the sediment core from the SML is characterized by δ 13 C about –59‰, which corresponds very closely to the δ 13 C of the CH 4 in the open water of the SML ranging from −62‰ to −58‰ (Figs. 4 and 5 both in ref. [6] ). Thus the δ 13 C values suggest that the CH 4 from the uppermost pore water in the sediment of the SML is the source of the CH 4 in the open water and do not indicate a reduction of the δ 13 C expected in case of substantial CH 4 production. Re-evaluation of the analysis of Günthel et al. [5] : data from Lake Stechlin Günthel et al. [5] underestimated the sediment flux and overestimated the emissions in Lake Stechlin and thus overestimated NOM (see below). We therefore re-evaluated the mass balances from Lake Stechlin to provide NOMC that are presented in Fig. 1 (see also Supplementary Table 3 in Supplementary Note 3.2 ). Oxic methanogenesis in Lake Stechlin was determined by Günthel et al. [5] using the same mass balance approach as in Lake Hallwil, but the sediment flux was estimated from a mesocosm experiment that involved two mesocosms. CH 4 surface fluxes from the two mesocosms were utilized to calculate CH 4 production within the mesocosms. Assuming that CH 4 production in the SML of the lake is the same as in the mesoscosm, F sed was determined by closing the mass balance of the SML in the lake. However, F surf from the mesocosms was overestimated because the gas transfer coefficient k 600 (transfer coefficient of CO 2 at 20 °C) determined for the open water of the lake was also used for the mesocosms [5] . The turbulence in the mesocosm is substantially lower than in the open water, i.e., in the uppermost 1 m of measurements the energy dissipation ε in the lake is 5–10 times larger than in the mesocosm (for details, see Supplementary Note 3.1 ; values on energy dissipation ε are from the data source of Supplementary Fig. 8 in Günthel et al. [5] ). Because k 600 ~ ε ¼ [12] , [13] , [14] , the difference in energy dissipation between lake and mesocosm suggest that k 600 in the mesocosm should be scaled by 5 − ¼ to 10 −¼ and is therefore only 67 or 56%, respectively, of the k 600 in the lake (see Supplementary Note 3.1 ). Hence, F surf in the mesocosm is only 67 or 56% of the value used by Günthel et al. [5] and the lower and upper bounds of the sediment flux become F sed = 1.8 and 2.0 mmol m −2 day −1 , respectively (Supplementary Table 2 and Supplementary Note 3.1 ) and thus are substantially larger than F sed = 1.4 mmol m −2 day −1 used by Günthel et al. [5] . The sediment flux derived from the mesocosm experiments conducted in the South Basin of Lake Stechlin in 2014 was also used for the stratified periods in 2016 and 2018 and in both basins of Lake Stechlin [5] . Hence the underestimation of the sediment flux in 2014 resulted in an overestimation of net production of CH 4 in all results of Günthel et al. [5] . NOMC calculated from the mass balance in the South and North Basin of Lake Stechlin, using the sediment fluxes corrected for the difference in turbulence between lake and mesocosms, are lower than 40% and agree well between 2014 and 2016 and between the basins (Supplementary Table 3 and detailed analysis in Supplementary Note 3.2 ). Hartmann et al. [11] collected in 2017 one sediment core from the SML in the South Basin of Lake Stechlin and provided another wind model for k 600 . Re-analysis of the CH 4 pore water of the sediment core provides a sediment flux into the water of 0.08–0.26 mmol m −2 day −1 (Supplementary Note 3.3 ) This flux is exceptionally low and incompatible with the sediment flux derived from the mesocosm experiments for the same basin, suggesting that the flux estimate based on a single sediment core is not representative for the average F sed in the SML. NOMC derived from this sediment flux and the model of k 600 of ref. [11] is exceptionally high (Fig. 1 , Supplementary Table 4 , and Supplementary Note 3.3 ). However, in addition to our re-analysis of the data of ref. [5] for Lake Stechlin, there is further evidence that NOMC is typically not very large in Lake Stechlin. According to Fig. 3 in Günthel et al. [5] , oxic CH 4 production was small in 2018 and even negative in the South Basin, implying NOMC < 0. Apparently, net oxidation instead of net production of CH 4 was the dominant process in the South Basin in 2018. Furthermore, in the central mesocosm (central reservoir) in Lake Stechlin, which was disconnected from the littoral CH 4 source for a very long time period, CH 4 concentrations were very low and close to atmospheric saturation [5] . Emissions from this mesocosm were therefore very small [5] showing no indication of significant in situ production of CH 4 . The mesocosms used for estimating oxic methanogenesis in Lake Stechlin were measured within 10 days after their filling and possibly had not reached steady state. Re-evaluation of the analysis of Günthel et al. [5] : data of DelSontro et al. [7] from additional lakes Günthel et al. [5] re-analyzed data from 7 lakes originally investigated by DelSontro et al. [7] and claim that in these lakes oxic methane production contributes between 82 and 100% of the total CH 4 emissions. However, these values are incompatible with the average net production of 25% stated by DelSontro et al. [7] for their systems with positive net production. Furthermore, according to DelSontro et al. [7] net production was negative in 30% of their lakes suggesting that in these lakes 100% of the emitted CH 4 was provided by CH 4 fluxes from the littoral zone. One of these lakes with negative net production was Lake Champlain [7] , but Günthel et al. [5] claim that in this lake 100% of the emissions originate from oxic methane production. It is unclear how Günthel et al. [5] performed the analysis of the data of DelSontro et al. [7] (see Supplementary Note 4.1 for details). We therefore determined NOMC for all lakes studied by DelSontro et al. [7] (Figs. 1 , S4 , and S5 ; Tables 2 and S5 , and details in Supplementary Note 4.1 ). Table 2 Analysis of data of DelSontro et al. [7] for the 7 lakes investigated by Günthel et al. [5] . Full size table DelSontro et al. [7] compared observations of the spatial distribution of CH 4 and δ 13 C of CH 4 in the SML of lakes with results from numerical simulations and provided estimates on the contribution of net oxic methane production in relation to a reference condition without biological processes. Their numerical model [7] assumes steady state and includes as sources for emissions only the CH 4 flux from the littoral and net oxic CH 4 production. The total emission for the reference condition therefore corresponds to the total flux from the littoral, F litt,tot . Del Sontro et al. [7] analyzed the impact of biological processes as fractional increase or decrease, f biol , of the CH 4 concentrations relative to the reference condition without oxidation. Figure 4 and Supplementary Table 8 of ref. [7] provide values on f biol + 1, denoted here as R CH4 (see Supplementary Note 4.1 ). Assuming that CH 4,equ is negligible compared to the CH 4 concentrations in the SML, R CH4 can be interpreted as the ratio of the total CH 4 emission F surf,tot to the emission under reference conditions F litt,tot , thus R CH4 ≈ F surf,tot / F litt,tot = (NOM + F litt,tot )/ F litt,tot = NOM/ F litt,tot + 1. The ratio of NOM to F surf,tot is given by NOMC = ( R CH4 − 1)/ R CH4 (for details and further analyses, see Supplementary Note 4.1 ). DelSontro et al. [7] provided R CH4 for six of the seven lakes investigated by Günthel et al. [5] . In these 6 lakes, NOMC is <20% and is negative in Lake Champlain indicating dominance of oxidation in this lake, which is consistent with ref. [7] (Table 2 ). The results on NOMC suggest that net production of CH 4 is not the dominant source of the CH 4 emissions from the lakes investigated but fluxes of CH 4 from shallow water regions (Fig. 1 ). NOMC is <50% in all lakes except in the South Basin of Lake Stechlin in 2017 where NOMC is unrealistically high because the average F sed in the SML is most likely substantially underestimated (the average F sed used by, e.g., Günthel et al. [5] for this basin in 2014, 2016, and 2018 was 5–18 times larger than F sed used for 2017, see Supplementary Note 3.3 ). On average NOMC is 10% (mean of all lakes using for Lake Stechlin the upper limits of 2016, i.e., 37 and 33%, for South and North Basin, respectively) and is 16% for the 6 lakes with lowest A sed / V SML . NOMC does not significantly increase with A surf or A sed / V SML (correlation using the same data as for the mean of all lakes: R 2 = 0.005, p = 0.8, and R 2 = 0.07, p = 0.3, respectively). Hence, there is no support for the hypothesis that net oxic CH 4 production contributes a major fraction of the CH 4 emitted from the lakes investigated or increases in importance with increasing lake size or decreasing A sed /V SML . The latter even suggests that NOMC is negligible. However, the results of our analysis cannot be taken as proof that NOM is negligible or, in contrast, as a confirmation that NOM contributes up to 37% to CH 4 emissions, because the uncertainty of the estimated NOMC is high: assessing the relevance of oxic methanogenesis from mass balance approaches involves the difference of comparative large contributions, i.e., surface emissions and sediments fluxes, which both have a large uncertainty. In particular, basin-wide average sediment fluxes from the littoral are not well constraint by estimates based on a single sediment core as in Lake Hallwil and Lake Stechlin, which becomes obvious from the comparison of sediment fluxes in the South Basin of Lake Stechlin derived from mesocosm experiments and the CH 4 pore water technique applied to a single core (Fig. 1 , data from ref. [11] , and Supplementary Note 3.3 ). Furthermore, closing mass balances of CH 4 requires that the components of the mass balance are measured at the same temperature, because CH 4 fluxes are temperature dependent [15] , and at the same time and not several months or even years apart as in Donis et al. [6] and Günthel et al. [5] , respectively. The investigations of Encinas Fernadez et al. [8] , DelSontro et al. [7] , and Peeters et al. [9] are based on the spatial distribution of CH 4 and consistently show that the observed horizontal distribution patterns of CH 4 in the SML require a large source of CH 4 in the shallow water region to explain the typically enriched concentrations in near shore zones. Spatially averaged CH 4 concentrations in the SML are not correlated with A surf but with A sed / A surf [8] implying that total emissions are proportional to A sed in the SML and that the littoral zone must therefore be an important source of CH 4 emissions [8] . The seasonal change in the horizontal distribution pattern of CH 4 in the SML and of the overall emission of CH 4 can be explained by a temperature-dependent sediment flux [9] . However, the quantification of sediment fluxes and of net CH 4 production using inverse modeling of spatial distributions of CH 4 [7] , [9] requires estimates of horizontal turbulent diffusion coefficients, which are unfortunately highly uncertain. Combining inverse modeling of spatial distributions, isotope measurements, and full mass balance approaches is not only a promising avenue to further constrain the relevance of oxic methanogenesis in lakes but also requires information on sediment fluxes, which appear to be the most uncertain component in the studies so far. Global emissions from lakes are dominated by emissions from small- and medium-sized lakes. Lakes with A surf < 1 km 2 contribute ~84% and lakes with A surf > 1 km 2 only ~16% of the global diffusive CH 4 emissions from lakes (Supplementary Table 1.2. in ref. [16] ). The contribution of oxic methanogenesis to global diffusive CH 4 emissions therefore depends on NOMC in small- and medium-sized lakes rather than on NOMC in large lakes. There seems to be consensus that diffusive emissions from lakes <1 km 2 are dominated by fluxes from littoral zones. Hence, improving the understanding and quantification of the sources of CH 4 in littoral zones appears to be particularly important for predicting the impact of changing conditions in lakes on the global CH 4 budget.